Tet-mediated covalent labelling of 5-methylcytosine for its genome-wide detection and sequencing 5-methylcytosine is an epigenetic mark that affects a broad range of biological functions in mammals. The chemically inert methyl group prevents direct labelling for subsequent affinity purification and detection. Therefore, most current approaches for the analysis of 5-methylcytosine still have limitations of being either density-biased, lacking in robustness and consistency, or incapable of analysing 5-methylcytosine specifically. Here we present an approach, TAmC-Seq, which selectively tags 5-methylcytosine with an azide functionality that can be further labelled with a biotin for affinity purification, detection and genome-wide mapping. Using this covalent labelling approach, we demonstrate high sensitivity and specificity for known methylated loci, as well as increased CpG dinucleotide coverage at lower sequencing depth as compared with antibody-based enrichment, providing an improved efficiency in the 5-methylcytosine enrichment and genome-wide profiling. DNA methylation (5-methylcytosine, 5mC) is a widely studied epigenetic mark. It is catalysed and maintained by a family of DNA methyltransferases in eukaryotes, and takes place at ~3–6% of the total cytosines in human genomic DNA [1] . DNA methylation could impact a broad range of biological processes in mammals, including gene expression, maintenance of genome integrity, parental imprinting, X-chromosome inactivation and development [2] , [3] , [4] . Moreover, abnormal DNA methylation has been associated with various human diseases, in particular cancers [5] , [6] , [7] . Knowledge of DNA methylation patterns and distributions in the genome is clearly crucial for us to understand the biological role of 5mC in normal human biology and aetiology of diseases. To date, three different strategies have been developed to profile and analyse genome-wide DNA methylation patterns (methylome) in eukaryotic cells [8] . Restriction enzyme-based approaches were the earliest strategy to be adapted for genome-wide methylation analysis. With the use of restriction enzymes that are sensitive to DNA methylation at the recognition sequence, 5mC could be detected at selected sequences. However, these approaches are limited to the specific restriction sites in the genome. In the second strategy, DNA fragments containing 5mC are enriched using affinity-based capture, including the use of 5mC-binding proteins (MBD-Seq) and antibody-based approaches (for example, methylated DNA immunoprecipitation or MeDIP-Seq). Bisulphite sequencing is the third common strategy in which denatured DNA is treated with sodium bisulphite, such that non-modified cytosine is converted to uracil, whereas methylated cytosine is left intact, thus allowing for base-resolution detection of cytosine methylation. Bisulphite sequencing is the current “gold standard” for DNA methylation analyses, owing to its sensitivity, high resolution and quantitativeness. However, this strategy cannot distinguish 5mC from 5hmC [9] , [10] , which was recently discovered as yet another form of cytosine methylation along with formyl-C (5fC) and carboxy-C (5caC) [11] , [12] . As a result, new approaches have been developed recently to distinguish 5hmC from 5mC with a single-base resolution [13] , [14] . Although whole-genome bisulphite sequencing approaches have been developed [15] , [16] , [17] and are increasingly adopted, affinity-based approaches, such as MBD-Seq and MeDIP-Seq, are still widely used, because of the low cost, in laboratories for genome-wide and loci-specific detection and/or profiling of 5mC. However, existing approaches commonly exhibit methylcytosine density-dependent bias that leads to lack of information at hypomethylated CpGs and non-CpG-methylated regions [18] , [19] , [20] . Bisulphite sequencing, although providing the most accurate methylation information, can be costly and requires a relatively large amount of samples because of DNA degradation during bisulphite treatment. As a result, further technology development of a robust, efficient, unbiased approach for whole-genome methylation profiling is still highly desirable. The development of such an approach will aid the general community in consistent profiling of methylomes, and in developing disease-specific diagnoses as well as establishing biomarkers [21] , [22] . Here we propose a new approach inspired by the discovery that 5mC can be oxidized by the iron(II)/α-ketoglutarate (α-KG)-dependent dioxygenases, the Tet (Ten-eleven translocation) family proteins (Tet1, 2 and 3), to 5hmC, which can be further converted to 5fC and 5caC in genomic DNA of mammalian cells [11] , [12] , [23] , [24] , [25] . We and others have invented chemical-labelling approaches to selectively tag 5hmC with functional groups, such as biotin, for robust affinity enrichment and sequencing without sequence and modification density bias [26] , [27] . We envisioned that chemical labelling of 5hmC could be combined with Tet-mediated conversion of 5mC to 5hmC for a selective labelling of 5mC for genome-wide detection and profiling. In our new approach, we first protect 5hmC with a glucose, using T4 bacteriophage β-glucosyltransferase (β-GT)-mediated glucosylation of 5hmC, which is a quantitative reaction [26] . We then employ the mouse Tet1 catalytic domain (residues 1367–2039, named mTet1 here and after) to oxidize 5mC to 5hmC, and simultaneously trap the newly generated 5hmC by β-GT-mediated transfer of a modified glucose moiety (6-N 3 -glucose) to afford 6-N 3 -β-glucosyl-5-hydroxymethyl-cytosine (N 3 -5gmC) [26] . Utilizing Huisgen cycloaddition (click) chemistry, a biotin tag (or any chemical tag) is then installed through the azide group of N 3 -5gmC for selective, efficient and unbiased pulldown of the original 5mC-containing DNA fragments for detection and genome-wide profiling ( Fig. 1 ) [26] . We named this new approach as Tet-assisted 5mC sequencing (TAmC-Seq). We show, by applying TAmC-Seq to profile 5mC in several mouse and human cell lines, that TAmC-Seq provides a wider coverage of CpG-containing genomic regions and captures a larger fraction of methylated CpGs with much fewer reads and less density bias compared with other affinity-enrichment methods. 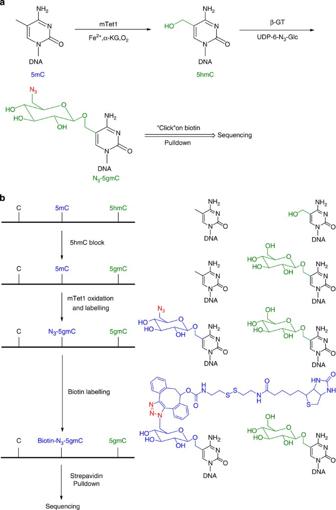Figure 1: Schematic diagram of the selective labelling of 5mC in DNA. (a) 5mC can be converted to 5hmC via mTet1-catalysed oxidation, and then labelled with a modified glucose moiety (6-N3-Glucose) by β-GT-mediated glucosylation to afford 6-N3-β-glucosyl-5-hydroxymethyl-cytosine (N3-5gmC), which could be further labelled using click chemistry. (b) The endogenous 5hmC in genomic DNA can be protected by glycosylation with regular glucose. Using a one-pot mTet1/β-GT protocol, 5mC is converted into N3-5gmC in the presence of both mTet1 and β-GT. The biotin moiety can then be installed for subsequent detection, affinity purification and sequencing. Figure 1: Schematic diagram of the selective labelling of 5mC in DNA. ( a ) 5mC can be converted to 5hmC via mTet1-catalysed oxidation, and then labelled with a modified glucose moiety (6-N 3 -Glucose) by β-GT-mediated glucosylation to afford 6-N 3 -β-glucosyl-5-hydroxymethyl-cytosine (N 3 -5gmC), which could be further labelled using click chemistry. ( b ) The endogenous 5hmC in genomic DNA can be protected by glycosylation with regular glucose. Using a one-pot mTet1/β-GT protocol, 5mC is converted into N 3 -5gmC in the presence of both mTet1 and β-GT. The biotin moiety can then be installed for subsequent detection, affinity purification and sequencing. Full size image Coupling Tet oxidation with β-GT for 5mC-specific labelling We cloned, expressed and purified mTet1 using a baculovirus expression system, according to the published procedure [24] . The enzyme activity was confirmed with in vitro activity assays (Methods and Supplementary Fig. S1 ) [13] . As indicated in the previous studies, the overall conversion of 5mC to 5fC/5caC by mTet1 is not processive in that the step of 5mC oxidation to 5hmC is kinetically faster than the subsequent 5hmC oxidation [12] . This knowledge presents an opportunity to capture the newly generated 5hmC with an efficient β-GT-mediated labelling reaction ( Fig. 1 ) [26] . We further confirmed that mTet1 could recognize and oxidize 5mC in a model double-stranded DNA (dsDNA) that contains hemi-5mC, full-5mC or hemi-5mC/hemi-5hmC modification ( Supplementary Fig. S2 ), ensuring that 5mC in various contexts in genomic DNA could be efficiently recognized and oxidized by mTet1 for further labelling. In addition, unlike TAB-Seq, which requires highly reactive mTet1 to fully convert 5mC to 5caC (ref. 13 ), most mTet1 proteins expressed from insect cells are fully active to convert 5mC to 5hmC in high efficiency. We tested our approach on a model dsDNA with a 5mC-containing 12mer oligonucleotide annealed to a complementary 16mer oligonucleotide containing a 5hmC modification ( Fig. 2a ). In the first step, we transferred a regular glucose from uridinediphosphoglucose to the 5hmC base using β-GT. The resulting 5gmC can no longer be oxidized or labelled as indicated, by treating the dsDNA with mTet1 under oxidation conditions ( Fig. 2a ). However, mTet1 oxidation efficiently converts the 5mC on the opposite strand to 5hmC. To avoid the potential overoxidation of 5mC to 5fC and 5caC by mTet1, we developed a one-pot procedure (referred to as the one-pot mTet1/β-GT reaction), envisioning that the 5hmC generated from oxidation of 5mC could be immediately captured and labelled with 6-N 3 -glucose by β-GT-mediated glucosylation, which could effectively prevent overoxidation of the newly generated 5hmC. The new N 3 -5gmC is then labelled with biotin via click chemistry. As shown in Fig. 2b , ~90% hemi-5mC on the model dsDNA could be successfully labelled with biotin in the one-pot mTet1/β-GT reaction, whereas the sequential treatment of the same dsDNA with mTet1 and then β-GT only afforded ~20% of the labelling ( Supplementary Fig. S3 ). 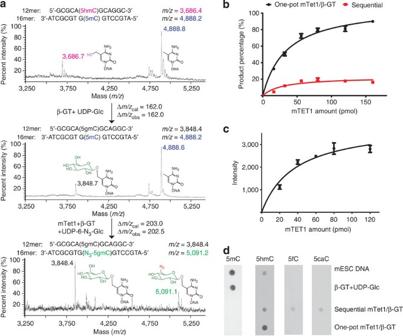Figure 2: Validation of the 5mC-labelling approach using model dsDNA and genomic DNA. (a) Mass spectrometry characterization of the model reaction with a 5mC containing a 5hmC-containing 12mer DNA, annealed to a 5mC-containing 16mer DNA. The reactions were monitored by matrix-assisted laser desorption/ionization–time of flight with the calculated molecular weight and observed molecular weight indicated. (b) Comparison of the 5mC conversion and labelling by using the one-pot mTet1/β-GT method (black curve) and sequential mTet1/β-GT method (red curve). 32mer dsDNA (50 pmol) containing a single 5mC was used as the substrate, and various concentrations of recombinant mTet1 were used as indicated. The conversion ratio was evaluated by dot blot assay of the attached biotin. As shown in the figure, the one-pot mTet1/β-GT method labelled over 90% of 5mC in the model DNA. Error bars represent data with s.d. from triplicate experiments. (c) 5mC labelling on mESC genomic sample by using the one-pot mTet1/β-GT method. Various concentrations of recombinant mTet1 were used as indicated. mTet1 protein (80–120 pmol) labelled most 5mC in 1 μg genomic DNA. Error bars represent data from triplicate experiments. (d) The labelled genomic DNA (mESC) products were validated by using antibodies against 5mC (1 μg), 5fC (150 ng) and 5caC (150 ng), and dot blot assay for 5hmC (150 ng). The one-pot mTet1/β-GT method converted most 5mC to 5hmC for subsequent labelling, with no overoxidation products detected. Figure 2: Validation of the 5mC-labelling approach using model dsDNA and genomic DNA. ( a ) Mass spectrometry characterization of the model reaction with a 5mC containing a 5hmC-containing 12mer DNA, annealed to a 5mC-containing 16mer DNA. The reactions were monitored by matrix-assisted laser desorption/ionization–time of flight with the calculated molecular weight and observed molecular weight indicated. ( b ) Comparison of the 5mC conversion and labelling by using the one-pot mTet1/β-GT method (black curve) and sequential mTet1/β-GT method (red curve). 32mer dsDNA (50 pmol) containing a single 5mC was used as the substrate, and various concentrations of recombinant mTet1 were used as indicated. The conversion ratio was evaluated by dot blot assay of the attached biotin. As shown in the figure, the one-pot mTet1/β-GT method labelled over 90% of 5mC in the model DNA. Error bars represent data with s.d. from triplicate experiments. ( c ) 5mC labelling on mESC genomic sample by using the one-pot mTet1/β-GT method. Various concentrations of recombinant mTet1 were used as indicated. mTet1 protein (80–120 pmol) labelled most 5mC in 1 μg genomic DNA. Error bars represent data from triplicate experiments. ( d ) The labelled genomic DNA (mESC) products were validated by using antibodies against 5mC (1 μg), 5fC (150 ng) and 5caC (150 ng), and dot blot assay for 5hmC (150 ng). The one-pot mTet1/β-GT method converted most 5mC to 5hmC for subsequent labelling, with no overoxidation products detected. Full size image Efficient and specific 5mC labelling in genomic DNA We first applied the established approach to label and profile genomic DNA from J1 mouse embryonic stem cells (referred to as mESC here and after). The candidate genomic DNA was sonicated into small fragments (~300–500 bp), and after protection of 5hmC with glucose, an appropriate amount of mTet1 was added to mediate 5mC oxidation. Using the one-pot mTet1/β-GT protocol, 80–120 pmol mTet1 converted and labelled most 5mC (cannot be detected by 5mC-specific antibody) to biotin from 1 μg genomic DNA with no overoxidized products (5fC and 5caC, detected by antibodies specific against these two bases) detected by immunoblot ( Fig. 2c ). In contrast, the sequential mTet1/β-GT treatment led to noticeable amounts of 5fC and 5caC generated ( Fig. 2d ). The conversion ratio of 5mC in mESC DNA is further confirmed by using liquid chromatography–mass spectrometry (LC–MS), which revealed that the endogenous 5hmC in genomic DNA were fully protected, and over 90% 5mC were converted and labelled to N 3 -5gmC ( Supplementary Fig. S4 and Supplementary Tables S1 and S2 ). Furthermore, we have also confirmed that the glucose labelling of 5hmC is not reversible under our assay conditions ( Supplementary Fig. S5 ) [28] . The biotin-labelled genomic DNA samples were subsequently processed by following the previously developed streptavidin pulldown protocol [29] . Application of TAmC-Seq for genome-wide 5mC profiling Previous comparison of approaches for mapping DNA methylation in ES cells highlighted the advantage of MeDIP-Seq for capturing a relatively large number of CpGs genome-wide, with relatively few reads, making this a cost-effective approach despite known biases associated with it [20] . Having established TAmC-Seq as both sensitive and specific for 5mC on model DNA, as well as its effectiveness on genomic DNA, we sought to further assess the utility of this new approach in determining the genome-wide distribution of 5mC. We therefore applied it to mESC genomic DNA. This experiment allowed further direct comparison of TAmC-Seq with previously published MeDIP-Seq [30] , and quantitative assessment of 5mC enriched by these two approaches. Comparison of read densities indicated that TAmC-Seq provides a highly similar pattern of enrichment as compared with MeDIP-Seq. Indeed, normalized count data in genome-wide bins (10 kb) displayed a correlation coefficient of 0.81 ( R 2 ) between TAmC-Seq and MeDIP-Seq ( Fig. 3a ). Likewise, read-normalized binary calling of methylated regions with increasing read-coverage thresholds (see Methods) showed that TAmC-Seq could account for >94% of the genomic sequences identified as methylated by MeDIP-Seq, with a minimum read depth of five, confirming the specificity of TAmC-Seq for capturing 5mC ( Fig. 3b ). The same regions were further validated by comparing with conventional whole-genome bisulphite sequencing data [13] , which revealed an average of 78.34% methylation at CpG dinucleotides ( Supplementary Table S3 ). We also found that TAmC-Seq generally exhibits a more even coverage than MeDIP-Seq ( Supplementary Figs S6 and S7 ). This observation suggests that, although specifically interrogating 5mC, TAmC-Seq is able to capture a larger fraction of methylated CpGs with reduced density-related bias, resulting in an effective spreading of reads more evenly throughout the methylated regions. 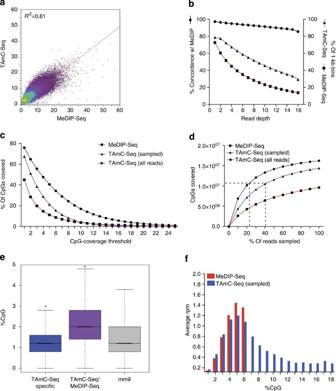Figure 3: Genome-wide comparison of MeDIP-Seq and TAmC-Seq. (a) Genome-wide correlation between TAmC-Seq and MeDIP-Seq (10 kb bins, reads per million). (b) Concordance and genomic coverage of TAmC-Seq and MeDIP-Seq with varying read depth thresholds. Percentage concordance (leftyaxis, black line), shows the percentage of 1 kb bins with the given read depth threshold in MeDIP-Seq that agree with TAmC-Seq. Rightyaxis shows the percentage of 1 kb bins covered at varying read depth thresholds per approach (TAmC-Seq, blue line; MeDIP-Seq, red line). Comparisons were performed using equal numbers of reads. (c) The fraction of CpGs covered genome-wide as a function of the depth of coverage for TAmC-Seq and MeDIP-Seq. TAmC-Seq reads were randomly sampled to match the number of reads in MeDIP-Seq. (d) The number of CpGs covered genome-wide by TAmC-Seq and MeDIP-Seq with varying fractions of reads used. The horizontal dotted line indicates 50% of all CpGs genome-wide. Vertical lines indicate the percentage of reads required to cover 50% of all CpGs (KCpG-Seq) with all TAmC-Seq reads or TAmC-Seq reads randomly sampled to match the number of MeDIP-Seq reads. (e) Mean %CpG content in TAmC-Seq-specific 1 kb bins, MeDIP-Seq/TAmC-Seq-concordant 1 kb bins and NCBI37v1/mm9; *P<0.0001,Z-test. (f) The distribution of 5mC signals (average reads per million, rpm) derived from MeDIP-Seq or TAmC-Seq for 1 kb bins stratified by %CpG content. Figure 3: Genome-wide comparison of MeDIP-Seq and TAmC-Seq. ( a ) Genome-wide correlation between TAmC-Seq and MeDIP-Seq (10 kb bins, reads per million). ( b ) Concordance and genomic coverage of TAmC-Seq and MeDIP-Seq with varying read depth thresholds. Percentage concordance (left y axis, black line), shows the percentage of 1 kb bins with the given read depth threshold in MeDIP-Seq that agree with TAmC-Seq. Right y axis shows the percentage of 1 kb bins covered at varying read depth thresholds per approach (TAmC-Seq, blue line; MeDIP-Seq, red line). Comparisons were performed using equal numbers of reads. ( c ) The fraction of CpGs covered genome-wide as a function of the depth of coverage for TAmC-Seq and MeDIP-Seq. TAmC-Seq reads were randomly sampled to match the number of reads in MeDIP-Seq. ( d ) The number of CpGs covered genome-wide by TAmC-Seq and MeDIP-Seq with varying fractions of reads used. The horizontal dotted line indicates 50% of all CpGs genome-wide. Vertical lines indicate the percentage of reads required to cover 50% of all CpGs ( K CpG-Seq ) with all TAmC-Seq reads or TAmC-Seq reads randomly sampled to match the number of MeDIP-Seq reads. ( e ) Mean %CpG content in TAmC-Seq-specific 1 kb bins, MeDIP-Seq/TAmC-Seq-concordant 1 kb bins and NCBI37v1/mm9; * P <0.0001, Z -test. ( f ) The distribution of 5mC signals (average reads per million, rpm) derived from MeDIP-Seq or TAmC-Seq for 1 kb bins stratified by %CpG content. Full size image To quantify the comparative efficiency of capture by each approach, we measured the number of CpG dinucleotides covered genome-wide as a function of the number of reads sequenced. With an equivalent number of reads, TAmC-Seq is capable of covering 22.4% more CpG dinucleotides than MeDIP-Seq (Fig. 3c ). When using the full set of TAmC-Seq reads, 76% of all CpGs were covered, approaching the estimated percentage of methylated cytosines observed in mouse ES cells (~80%) as determined by conventional bisulphite sequencing ( Fig. 3c ) [31] . As an overall measure of efficiency, we next determined the number of reads required to cover 50% of all CpG dinucleotides ( K CpG-Seq ), assuming that greater than this fraction are methylated in mouse ES cells [31] . K CpG-Seq for TAmC-Seq was 7.7 × 10 6 reads (~41% of total), whereas MeDIP-Seq failed to achieve 50% coverage with an equivalent number of reads ( Fig. 3d ). When utilizing the full set of TAmC-Seq reads (3.5 × 10 7 ), K CpG-Seq reached 22.7% ( Fig. 3d ). These results indicate that TAmC-Seq is able to enrich methylated CpGs more effectively than MeDIP-Seq, and demonstrate the increased efficiency of the approach for specifically interrogating 5mC. The primary drawback of the current affinity-based 5mC-enrichment procedures is that they often exhibit CpG density bias, which can vary depending on antibody/protein source and the concentration of salts used during immunoprecipitation and/or elution. As a chemical-based approach that takes advantage of covalent connection and the high-affinity biotin/streptavidin enrichment, TAmC-Seq offers the potential to reduce the impact of such variables. To compare the relative biases associated with TAmC-Seq and MeDIP-Seq, we first determined %CpG content within 1-kb bins concordant among each approach, as well as those captured specifically by TAmC-Seq, but not MeDIP-Seq, at read-coverage threshold of ≥5, representing 94% of MeDIP-Seq 1-kb bins ( Fig. 3e ). Indicative of enrichment for 5mC by both approaches, concordant regions have significantly higher %CpG content relative to the genome-wide mean ( P <0.0001, Z -test). However, at regions specific to TAmC-Seq, the CpG percentage content is significantly lower than the genomic mean ( P <0.0001, Z -test). This observation suggests that although TAmC-Seq captured a significant fraction of methylated regions detected by MeDIP-Seq, it also recovered additional loci with a lower percentage of CpG content. TAmC-Seq-specific regions were confirmed as methylated by comparing with the whole-genome bisulphite sequencing data [13] , [31] , showing 76.34% methylation of CpG dinucleotides ( Supplementary Table S3 ). To further examine the average 5mC signals generated by TAmC-Seq and MeDIP-Seq at regions with varying percentage of CpG content, we also stratified genome-wide 1 kb bin read counts (reads per million) by %CpG content. We found that TAmC-Seq is able to capture a wider range of CpG content than that of MeDIP-Seq, for which the distribution reflected the CpG content previously observed for MeDIP-Seq and MBD-Seq in mammalian genomes [20] , [32] ( Fig. 3f ). Together, these data demonstrate a high concordance between TAmC-Seq and MeDIP-Seq, with TAmC-Seq providing additional access into the methylome compared with MeDIP-Seq. Global comparison of methods that map DNA methylation Next, we further compared the performance of TAmC-Seq with MethylC-Seq and MeDIP-Seq, two common approaches for DNA methylation mapping. We performed TAmC-Seq in human mammary epithelial cells (HMEC) and the breast cancer cell line HCC1954, and compared these maps with those previously generated by bisulphite sequencing and MeDIP-Seq [33] , [34] . After mapping and PCR duplicate filtering, the number of usable reads from TAmC-Seq and MeDIP-Seq were comparable (TAmC HMEC =6.5 million, MeDIP HMEC =6.3 million, TAmC HCC1954 =7.1 million). Previously, using bisulphite sequencing, we had observed large domains of hypomethylation in HCC1954 compared with HMEC. This is clearly recapitulated by TAmC-Seq ( Fig. 4a ). At greater resolution, TAmC-Seq and bisulphite sequencing are also concordant; both approaches clearly reveal that the promoter of the DACH1 tumour suppressor is methylated, that the CpG island near the KLF5 promoter is unmethylated, and that KLF12 has an unmethylated CpG island but with methylated shores. 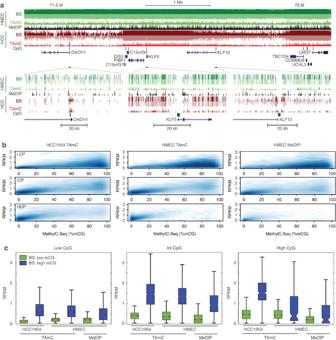Figure 4: Comparison of affinity approaches with bisulphite sequencing. (a) UCSC Genome Browser snapshots of TAmC-Seq, MeDIP-Seq and methylC-Seq near the DACH1 tumour suppressor locus. (b) Density plots of affinity enrichment compared with bisulphite sequencing at low CpG promoters (LCP, top), intermediate CpG promoters (ICP, middle) and high CpG promoters (HCP, bottom). (c) The distribution of affinity enrichment at promoters with low methylation (≤25% mCG, green) and high methylation (>75%, blue), as determined by bisulphite sequencing. Figure 4: Comparison of affinity approaches with bisulphite sequencing. ( a ) UCSC Genome Browser snapshots of TAmC-Seq, MeDIP-Seq and methylC-Seq near the DACH1 tumour suppressor locus. ( b ) Density plots of affinity enrichment compared with bisulphite sequencing at low CpG promoters (LCP, top), intermediate CpG promoters (ICP, middle) and high CpG promoters (HCP, bottom). ( c ) The distribution of affinity enrichment at promoters with low methylation (≤25% mCG, green) and high methylation (>75%, blue), as determined by bisulphite sequencing. Full size image We next compared the performance of the affinity-based approaches with bisulphite sequencing. One way to assess the relative performance is to compute the correlation of two assay results throughout the genome. We partitioned the genome into non-overlapping 10-kb bins, measured DNA methylation from both affinity approaches as RPKM (reads per million base pairs mapped per kb of model) and plotted DNA methylation levels relative to MethylC-Seq ( Supplementary Fig. S8 ). TAmC-Seq in HCC1954 reveals that the approach can recover global hypomethylation. Although the results for TAmC-Seq and MeDIP-Seq in HMEC cells are comparable, we observed a greater dynamic range in TAmC-Seq, which we discuss below. Although DNA methylation is found throughout the genome, its most recognized role is as a mark of gene repression when found at promoters. Thus, a key performance metric of any approach to map DNA methylation is the ability to distinguish methylated from unmethylated promoters. To assess this performance, we compared the two affinity-based approaches with MethylC-Seq at promoters, where promoters are partitioned by CpG content (L/I/H=low/intermediate/high) ( Fig. 4b ). For all three examples, we observed a positive correlation between affinity-based and bisulphite-based DNA methylation. For all classes of promoters in HMEC cells, TAmC-Seq correlated better with bisulphite sequencing than MeDIP-Seq (low CpG: R TAmC =0.18>0.15= R MeDIP ; intermediate CpG: R TAmC =0.67>0.49= R MeDIP ; high CpG: R TAmC =0.40>0.37= R MeDIP . Furthermore, in agreement with the global analysis above, it appears that the dynamic range of TAmC-Seq is greater than that of MeDIP-Seq. To quantify this observation, we examined the affinity enrichment for lowly methylated (%CpG≤25%) and highly methylated (%CpG>75%) promoters ( Fig. 4c ), as determined by bisulphite sequencing. We observe that the median level of TAmC-Seq enrichment is between 32.7 and 91.0% greater than that of MeDIP-Seq ( P high CpG =0.0035; P intermediate CpG =8.0E-47; P low CpG =1.1E-39, Wilcoxon rank sum test). These results suggest the TAmC-Seq dynamic range is greater than that of the MeDIP-Seq. To systematically compare the ability of TAmC-Seq and MeDIP-Seq to distinguish methylated from unmethylated promoters, we first focused on a curated set of promoters that are lowly or highly methylated in HMEC according to bisulphite sequencing. We identified 1,388 promoters that are consistently highly methylated (>75% mCG) within and around the CpG island/transcription start site (TSS) and 7,621 promoters that are consistently lowly methylated (≤25% mCG; Fig. 5a ). We then utilized a random forest to classify promoters as methylated or unmethylated, given only affinity enrichment. MeDIP-Seq gives a higher classification error rate than TAmC-Seq ( Fig. 5b ), indicating that TAmC-Seq enrichment is a better predictor of DNA methylation than the MeDIP-Seq enrichment. Extending this analysis to all promoters, we made similar observations ( Fig. 5c ). For all grades of CpG content, MeDIP-Seq consistently performs worse than TAmC-Seq for the task of classifying lowly and highly methylated promoters. 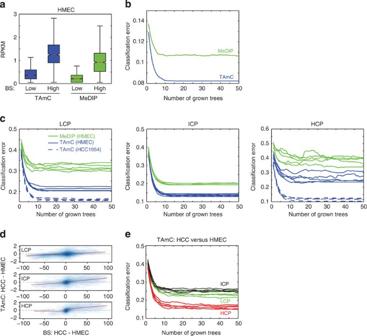Figure 5:Classification comparison of TAmC-Seq and MeDIP-Seq. (a) The distribution of TAmC-seq and MeDIP-seq enrichment for a set of curated promoters that are consistently highly methylated (>75% mCG) within and around the CpG island/TSS, or consistently lowly methylated (≤25% mCG). (b) Random forest classification error in distinguishing methylated from unmethylated curated promoters ina. (c) Random forest classification error in distinguishing methylated from unmethylated promoters, for different CpG densities. An equal number of methylated and unmethylated promoters were randomly sampled, and subsequently classified for each CpG density class. Each line represents a different random sampling of promoters. The high variance of HCPs is due to the small number of methylated high-CpG promoters in HMEC. (d) A density plot of bisulphite change (%mCG(HCC1954)—%mCG(HMEC)) compared with TAmC change (RPKM(HCC1954)—RPKM(HMEC)) for promoters of various CpG content. The red line is the lowest weighted curve; RPKM, reads per million base pairs mapped per kb of model. (e) Random forest classification error in distinguishing hypermethylated from hypomethylated promoters for different CpG densities. An equal number of hypermethylated and hypomethylated promoters were classified for each CpG density class. Each line represents a different random sampling of promoters. Figure 5: Classification comparison of TAmC-Seq and MeDIP-Seq . ( a ) The distribution of TAmC-seq and MeDIP-seq enrichment for a set of curated promoters that are consistently highly methylated (>75% mCG) within and around the CpG island/TSS, or consistently lowly methylated (≤25% mCG). ( b ) Random forest classification error in distinguishing methylated from unmethylated curated promoters in a . ( c ) Random forest classification error in distinguishing methylated from unmethylated promoters, for different CpG densities. An equal number of methylated and unmethylated promoters were randomly sampled, and subsequently classified for each CpG density class. Each line represents a different random sampling of promoters. The high variance of HCPs is due to the small number of methylated high-CpG promoters in HMEC. ( d ) A density plot of bisulphite change (%mCG(HCC1954)—%mCG(HMEC)) compared with TAmC change (RPKM(HCC1954)—RPKM(HMEC)) for promoters of various CpG content. The red line is the lowest weighted curve; RPKM, reads per million base pairs mapped per kb of model. ( e ) Random forest classification error in distinguishing hypermethylated from hypomethylated promoters for different CpG densities. An equal number of hypermethylated and hypomethylated promoters were classified for each CpG density class. Each line represents a different random sampling of promoters. Full size image Finally, having explored the performance of TAmC-Seq in each cell line independently, we next examined its performance across multiple samples by comparing HMEC with HCC1954. At promoters, changes of DNA methylation observed from TAmC-Seq are positively correlated with changes in absolute DNA methylation as measured by bisulphite sequencing ( Fig. 5d ). Employing a random forest to classify hypermethylated (%mCG HCC1954 —%mCG HMEC ≥50%) and hypomethylated (%mCG HCC1954 —%mCG HMEC ≤−50%) promoters, we found that TAmC-Seq approaches 75% accuracy for low- and intermediate-CpG promoters, and up to 85% accuracy for high CpG-content promoters (Fig. 5e ). This ability to gauge cell-type specific DNA methylation at promoters of varying CpG content indicates that TAmC-Seq performance is relatively sequence independent. In summary, affinity-based enrichment of methylated DNA, when coupled with high-throughput sequencing, offers an effective approach for assessing DNA methylation on the genomic scale. The development of 5mC-specific antibodies has made possible genomic DNA methylation profiling in various biological systems. However, the primary pitfall associated with 5mC immunoprecipitation is the methyl-CpG-density-dependent bias, which ultimately results in missing certain portions of the methylome. In addition, various factors could contribute to inconsistency of results obtained from antibody-based experiments. Here we report an enzymatic strategy to specifically modify the inert methyl group of 5mC, which utilizes a covalent linkage and a high-affinity biotin/streptavidin interaction to label and enrich 5mC in an unbiased manner. We found that TAmC-Seq is highly sensitive and specific to 5mC, and captures a larger fraction of CpG dinucleotides with far fewer reads than MeDIP-Seq. Furthermore, TAmC-Seq provides a wider range of access to genomic regions with varying CpG-dinucleotide frequencies, reducing CpG-density-dependent bias compared with that of MeDIP-Seq. In addition, the covalent strategy ensures the robustness of the approach for reliable profiling and/or loci-specific pulldown and interrogation of DNA methylation without resorting to the more costly bisulphite-sequencing approach. TAmC-Seq thereby offers a consistent and robust tool to facilitate effective enrichment and epigenomic profiling of DNA methylation. Recombinant mTET1 expression and purification The catalytic domain of Mouse Tet1 gene (GU079948) was cloned into Bss HII and Not I sites of the N-terminal Flag-tagged pFastBac Dual vector (Invitrogen) and expressed in Bac-to-Bac baculovirus insect cell expression system. The recombinant Flag-mTet1 (residues 1367–2039) was purified according to the published procedure (Supplementary Fig. S1a, b) [13] . Recombinant β-GT expression and purification The recombinant β-GT was expressed and purified following the previous protocol [26] . Oligonucleotide synthesis 12mer, 16mer, 32mer and 44mer oligonucleotides containing single CpG with modified cytosine (5mC or 5hmC) were prepared by incorporating the phosphoramidite (5mC and 5hmC) at the desired position during solid-phase synthesis. The reagents and phosphoramidites (5mC and 5hmC) were purchased from Glen Research. All synthetic oligonucleotides were further purified with denaturing polyacrylamide gel electrophoresis. The oligonucleotides containing normal bases were purchased from Operon. Synthesis of UDP-6-N 3 -UDP UDP-6-N 3 -UDP is synthesized by following the previous protocol [26] . Recombinant mTet1 in vitro activity assay Various concentration of recombinant mTet1 and 20 pmol 12/16mer dsDNA with internal 5-position methylated cytosine on 12mer DNA were added into the 20 μl reaction mixture containing 50 mM HEPES (pH 8) 75 μM Fe(NH 4 ) 2 (SO 4 ) 2 , 2 mM ascorbic acid and 1 mM α-KG for 1 h at 37 °C. The reaction products were then validated by matrix-assisted laser desorption/ionization–time of flight ( Supplementary Fig. S1c ). Anti-5mC antibody was obtained from Epigentek (Cat: A-1014). Antibodies against 5fC and 5caC were obtained from Active Motif (Cat: 61223 and 61225, respectively). Synthetic standards were used to quantify 5mC and 5hmC in activity assays [26] . Recombinant mTet1 substrate-selectivity assay mTet1 (20 pmol), β-GT (40 pmol) and 32/44mer (20 pmol) dsDNA with desired modified cytosine (C, 5mC or 5hmC) were added into the 30 μl reaction mixture containing 50 mM HEPES (pH 8), 75 μM Fe(NH 4 ) 2 (SO 4 ) 2 , 2 mM ascorbic acid, 1 mM α-KG, 10 mM MgCl 2 , 1 mM dithiothreitol and 100 μM UDP-6-N 3 -Glucose for 1 h at 37 °C. The DNA products were then purified using Qiagen DNA purification kit, and subsequently mixed with 150 μM Dibenzylcyclooctyne-Fluor (Click Chemistry Tools Bioconjugate Technology Company) for 2 h at 37 °C. The labelled products were purified with the Qiagen purification kit, and 200 ng was loaded to 16% urea-denatured acrylamide gels to separate the annealed strands. The gel was first scanned under 563 nm and the fluorescence was detected at 582 nm, and then stained with Syber Green ( Supplementary Fig. S2 ). Recombinant mTet1- and β-GT-based chemical labelling of DNA β-GT (40 pmol) and 3 μg sonicated mESC genomic DNA were added into the 30 μl reaction mixture containing 50 mM HEPES (pH 8), 25 mM MgCl 2 and 300 μM UDP-Glucose for 1 h at 37 °C. The product was purified using the Qiagen DNA purification kit. Subsequently, 160 pmol mTet1, 80 pmol β-GT and 2 μg treated genomic DNA were added into the 50 μl reaction mixture containing 50 mM HEPES (pH 8), 75 μM Fe(NH 4 ) 2 (SO 4 ) 2 , 2 mM ascorbic acid, 1 mM α-KG, 10 mM MgCl 2 , 1 mM dithiothreitol and 150 μM UDP-6-N 3 -Glucose for 1 h at 37 °C. The DNA product was then purified and directly used in click reaction. Huisgen cycloaddition reaction and pulldown The Huisgen cycloaddition (click) reaction and pulldown was processed according to the previous protocol [26] ( Supplementary Methods ). Quantitative analysis of 5mC oxidation using L–-MS/MS mESC genomic DNA (1 μg) with different treatment protocols (as indicated) was digested by using nuclease P1 (2U) in 30 μl of buffer containing 25 mM of NaCl and 2.5 mM of ZnCl 2 at 37 °C for 2 h, followed by the addition of NH 4 HCO 3 (1 M, 3 μl) and Venom phosphodiesterase (0.001 U) and 2 h incubation at 37 °C. After an additional incubation at 37 °C for 2 h with alkaline phosphatase (0.5 U), the solution was diluted twofold, and 10 μl of the solution was injected into LC–MS/MS. The nucleosides were separated by reverse-phase ultra-performance LC on a C18 column, with online MS detection using Agilent 6410 QQQ triple-quadrupole LC mass spectrometer in a positive electrospray ionization mode. The nucleosides were quantified using the nucleoside to base ion mass transitions. Quantification was performed by comparison with the standard curve obtained from pure nucleoside standards running at the same batch of samples. The ratio of 5mC oxidation was calculated based on the calculated concentrations ( Supplementary Fig. S4 ). Stability assay of glucosylated 5hmC using model dsDNA β-GT (40 pmol) and 9/11mer (400 pmol) model dsDNA containing a single 5hmC were added into a 30-μl reaction mixture containing 50 mM HEPES (pH 8), 25 mM MgCl 2 and 300 μM UDP-glucose for 1 h at 37 °C. The product with glucosylated 5hmC was purified using the Qiagen DNA purification kit. Subsequently, 40 pmol β-GT and 200 pmol product DNA were added into a 30 μl reaction mixture containing 50 mM HEPES (pH 8), 25 mM MgCl 2 and 1 mM UDP for 1 h at 37 °C. The reactions were monitored by matrix-assisted laser desorption/ionization–time of flight, with the calculated molecular weight and observed molecular weight indicated ( Supplementary Fig. S5 ). No 5hmC was observed, thus indicating that the reaction is not reversible under the assay conditions we typically employed for TAmC-Seq. TAmC-Seq library generation 5mC-enriched-genomic DNA (25 ng) from three independent 5mC captures or one non-enriched input genomic DNA was end-repaired, adenylated and ligated to an Illumina Genomic DNA Adapters (Genomic DNA adapter oligo mix), according to standard Illumina protocols for ChIP-Seq library construction, maintaining the proper molar ratios of the adapter to insert. Adapter-ligated fragments ~200–350 bp were gel-purified by 2% agarose gel electrophoresis and PCR-amplified for 18 PCR cycles. Libraries were checked for quality and quantified using an Agilent 2100 Bioanalyzer DNA 1000 Chip. TAmC-Seq library sequencing and read processing TAmC-Seq libraries were sequenced using the Illumina HiScan platform. Cluster generation was performed with Illumina TruSeq cluster kit v2-cBot-HS. Single reads 51-bp sequencing was completed with Illumina TruSeq SBS kit v3-HS. A dedicated PhiX control lane, as well as 1% PhiX spike in all other lanes, was used for automated matrix and phasing calculations. Image analysis and base calling were performed with the standard Illumina pipeline. FASTQ sequences were aligned to NCBIv1/mm9 with Bowtie v0.17.2 retaining non-duplicate, unique matches to the genome with no more than three mismatches in the first 30 bases. For binned analyses, unique non-duplicate reads from replicate 5mC captures were concatenated, extended to a length of 200 bp in the direction of the read, counted in 1 or 10 kb bins, and normalized to the total number of reads in millions. The total number of unique, non-duplicate reads obtained from each replicate experiment and the total number of unique, non-duplicate reads from each approach are listed in Supplementary Table S4 . In cases where the number of reads from TAmC-Seq and MeDIP-Seq were normalized before analysis, reads were randomly sampled from the larger TAmC-Seq set to match the number of reads in the MeDIP-Seq set. MeDIP-Seq data and read processing Previously published MeDIP-Seq reads [30] were downloaded from the ENA Short Read Archive (accessions ERR031627 and ERR031630) and the DDBJ Read Archive (accession DRA000030). As reads from both MeDIP-Seq and TAmC-Seq are tags representing larger DNA fragments, and the MeDIP-Seq reads were derived from paired-end sequencing experiments (although TAmC-Seq reads were derived from a single-read experiments), only read one from the MeDIP-Seq data were used for analyses. Thirty-six base pair MeDIP-Seq reads were aligned to NCBIv1/mm9, extended to a length of 200 bp and post processed in an identical manner, parallel with TAmC-Seq sequences as described above. TAmC-Seq versus MeDIP-Seq concordance analysis Binned data (1 kb) were thresholded by the number of read counts in MeDIP-Seq and TAmC-Seq (randomly sampled to match MeDIP-Seq read counts). Bins at or above defined thresholds were extracted for each capture approach and the number of bins in common was determined. For each 5mC capture approach, the percentage of total 1 kb bins genome-wide was also tracked at each threshold. Comparison with conventional whole-genome bisulphite sequence data was done using CpG methylation signals only (5mC+5hmC) derived as previously published as part of ref. 13 with sequence data from ref. 27 (NCBI GEO accession GSE30206). The HMEC and HCC1954 bisulphite sequencing data were also obtained from GEO (accession GSE29069). CpG-coverage analysis Genomic positions for each CpG dinucleotide were derived for the genome (NCBIv1/mm9), and the number of post-processed MeDIP-Seq or TAmC-Seq reads covering each CpG were counted. Both the number of CpGs covered and the depth of coverage were tracked. For determining K CpG-Seq , fractions of MeDIP-Seq and TAmC-Seq reads were randomly and progressively sampled at 10% intervals up to 100% of reads. The percentage/number of reads required to cover 50% of all CpG dinucleotides, assuming greater than this number are methylated, is defined as K CpG-Seq . CpG-content analysis For determining %CpG content in concordant and discordant 1 kb bins, a read threshold of 5 was used, using an equivalent number of MeDIP-Seq and randomly sampled TAmC-Seq reads. Bins specific to TAmC-Seq at or above this threshold were identified as discordant, whereas concordant bins were those in common between MeDIP-Seq and TAmC-Seq. The mean %CpG content in a set of 1 kb bins was determined and compared with the genome-wide average using a Z -test. For determining 5mC signals with varying %CpG content, 1-kb bin read counts (reads per million) were determined genome-wide, and bins were subsequently stratified by %CpG content at 1% intervals, from 1 to 18%. The mean reads per million for all 1 kb bins with a given %CpG content was then determined for MeDIP-Seq and TAmC-Seq. Comparative analyses of methods that map DNA methylation Random forest classification was performed using Matlab (function TreeBagger, OOBPred=on). How to cite this article: Zhang, L. et al . Tet-mediated covalent labelling of 5-methylcytosine for its genome-wide detection and sequencing. Nat. Commun. 4:1517 doi: 10.1038/ncomms2527 (2012).